Cryptochromesare critical for the development of coherent circadian rhythms in the mouse suprachiasmatic nucleus Cryptochrome ( Cry ) 1 and Cry2 are regarded as critical components for circadian rhythm generation in mammals. Nevertheless, cultured suprachiasmatic nucleus (SCN) of neonatal Cry double deficient ( Cry1 −/− /Cry2 −/− ) mice exhibit circadian rhythms that damp out in several cycles. Here, by combining bioluminescence imaging of Per1-luc and PER2::LUC with multielectrode recording, we show developmental changes in SCN circadian rhythms in Cry1 −/− /Cry2 −/− mice. At the tissue level, circadian rhythms are found in neonatal but not in adult SCN, whereas at the cellular level, rhythms are detected in both SCN. Cellular circadian rhythms are synchronized in neonates, but not in adults, indicating a loss of rhythm synchrony in the course of development. Synchronized circadian rhythms in adult Cry1 −/− /Cry2 −/− SCN are restored by coculture of neonatal, but not of juvenile, SCN. These findings indicate that CRY1 and CRY2 are necessary for the development of intercellular networks that subserve coherent rhythm expression in adult SCN. Mammalian circadian rhythms in physiology and behaviour are regulated by a central clock located in the hypothalamic suprachiasmatic nucleus (SCN) [1] . It is widely accepted that the circadian oscillation is generated by an autoregulatory transcription and translation feedback loop consisting of the clock genes, Period ( Per ) 1 , Per2 , Cryptochrome ( Cry ) 1 , Cry2 , Bmal1 and Clock , and their protein products [2] . Cry1 and Cry2 double deficient ( Cry1 −/− /Cry2 −/− ) mice exhibit aperiodic behaviours immediately after transfer from light–dark cycles (LD) to constant darkness (DD) [3] . In addition, rhythmic clock gene expression [4] and neural activity [5] are absent in the SCN of Cry1 −/− /Cry2 −/− mice housed in DD. The 24-h rhythms observed in behaviour [3] and clock gene expression [6] in LD are interpreted to be driven extrinsically by light [3] . Nevertheless, some Cry1 −/− /Cry2 −/− mice begin activity before dark onset in LD [7] , [8] . Such pre-dark activities cannot be explained by extrinsic light effects and may reflect an underlying self-sustained circadian rhythm [7] . Recently, robust circadian rhythms of PER2::LUC were demonstrated at the single-cell level and at the tissue level of cultured SCN from neonatal Cry1 −/− /Cry2 −/− mice [9] . The tissue-level PER2::LUC rhythms damped out in several cycles but were restored by coculture with a wild-type (WT) SCN, suggesting that a diffusible factor(s) supports synchrony of the SCN [9] . We also reported that the spontaneous neuronal firing in cultured SCN of neonatal Cry1 −/− /Cry2 −/− mice is rhythmic [10] . These findings are inconsistent with previous reports demonstrating a loss of circadian rhythms in clock gene expressions at both the cell [11] and tissue [12] levels of the cultured SCN in Cry1 −/− /Cry2 −/− mice. The discrepancy could be due to differences in the measures used [11] and/or the age of animals [12] . The dual roles of cellular couplings in the SCN are emphasized in the expression of circadian rhythms: synchronization and reinforcement of the cellular circadian rhythms [11] , [13] . There is some evidence that the cellular coupling in the SCN differs between neonatal and adult mice. For example, responses of gene expression rhythms to medium exchange [14] and tetrodotoxin (TTX) [11] , [15] , a sodium channel blocker, are greater in the neonatal SCN than in the adult. In vivo , the neonatal SCN is more sensitive to non-photic time cues than the adult SCN, as highlighted by the entrainment to maternal rhythms [16] , [17] . These findings suggest that the cellular coupling that allows rhythm synchrony in the SCN changes during postnatal development. However, the mechanisms of cellular couplings are still poorly understood. During pre- and postnatal development, the SCN changes physiologically and morphologically. The numbers of synapses and astrocytes increase rapidly during the early developmental period, and apoptotic neuronal death occurs in the SCN from the late embryonic days through postnatal day 6 (P6) (refs 18 , 19 ). Furthermore, immunostained calcium-binding protein in the SCN decreases during the postnatal period [20] . These changes may influence the cell networks of the SCN, and alter the cellular couplings for rhythm synchrony. In the present study, we aim to understand roles of CRYs in the expression of SCN circadian rhythms in different physiological functions and at different stages of postnatal development. Taking advantage of luciferase reporters ( Per1-luc , PER2::LUC), we examined the circadian rhythms of Per1 expression and intracellular PER2 at the single-cell as well as tissue levels in cultured SCN of Cry1 −/− /Cry2 −/− mice through the course of development. We also monitored spontaneous neuronal firing in the cultured SCN using a multielectrode array dish (MED) system. Surprisingly, circadian rhythms at the SCN cell level were detected from the neonatal stage to adulthood, while the rhythms at the SCN tissue level were observed only in the early postnatal period. Circadian rhythms of Per1-luc seemed to be more sensitive to CRY double deficiency than that of PER2::LUC. Coculture of neonatal Cry1 −/− /Cry2 −/− SCN restored circadian PER2::LUC rhythms at the tissue level in the adult SCN of Cry1 −/− /Cry2 −/− mice. These findings indicate that CRY1 and CRY2 are dispensable for circadian rhythm generation, but necessary for the development of cellular couplings for rhythm synchrony, which are crucial for expression of coherent circadian rhythms in adult SCN. Developmental changes in circadian rhythms of Per1 and PER2 Developmental changes of circadian rhythms in Per1-luc and PER2::LUC were examined in the cultured SCN of Cry1 −/− /Cry2 −/− mice. Marked differences were detected in the circadian rhythms at the SCN tissue level between the Cry1 +/+ /Cry2 +/+ (control) and Cry1 −/− /Cry2 −/− mice during postnatal development ( Fig. 1 ). 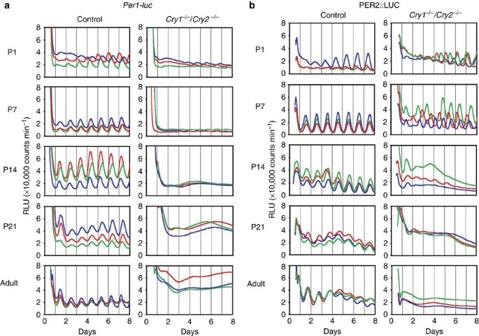Figure 1: Developmental changes in circadian rhythms ofPer1-lucand PER2::LUC at the SCN tissue level. Circadian rhythms at different stages of development are illustrated inPer1-luc(a) and PER2::LUC (b) from the control (left) andCry1−/−/Cry2−/−mice (right). Representative results from three littermates are demonstrated in each panel with different colours. The ages of mice at harvest are indicated at the left margin; the number of days in culture is indicated on the abscissa with day 0 as the day of harvest. The ordinate indicates the intensity of bioluminescence in relative light units (RLUs). The vertical lines in panels indicate a local time of 0000, hours. The variability of circadian peak phase in individual rhythms was calculated in PER2::LUC rhythm on the 2nd culture day. The variability was not different between the SCN of the control andCry1−/−/Cry2−/−mice harvested at P1, but significantly larger in the SCN ofCry1−/−/Cry2−/−mice (s.d.; 4.4 h,n=6) than in the control (s.d.; 0.3 h,n=4) harvested at P7. Figure 1: Developmental changes in circadian rhythms of Per1-luc and PER2::LUC at the SCN tissue level. Circadian rhythms at different stages of development are illustrated in Per1-luc ( a ) and PER2::LUC ( b ) from the control (left) and Cry1 −/− /Cry2 −/− mice (right). Representative results from three littermates are demonstrated in each panel with different colours. The ages of mice at harvest are indicated at the left margin; the number of days in culture is indicated on the abscissa with day 0 as the day of harvest. The ordinate indicates the intensity of bioluminescence in relative light units (RLUs). The vertical lines in panels indicate a local time of 0000, hours. The variability of circadian peak phase in individual rhythms was calculated in PER2::LUC rhythm on the 2nd culture day. The variability was not different between the SCN of the control and Cry1 −/− /Cry2 −/− mice harvested at P1, but significantly larger in the SCN of Cry1 −/− /Cry2 −/− mice (s.d. ; 4.4 h, n =6) than in the control (s.d. ; 0.3 h, n =4) harvested at P7. Full size image Significant circadian rhythms of Per1-luc expression were detected at all ages examined in the control, but only during the early postnatal period (P1 and P7) in Cry1 −/− /Cry2 −/− mice ( Fig. 1a ). Circadian amplitudes determined at 5th culture day of each preparation increased after birth, peaked at P7–P14 and declined afterwards in the control mice ( Supplementary Fig. S1a ). The amplitudes in Cry1 −/− /Cry2 −/− mice were significantly lower than those in the control at P1 and P7, and undetectable at P14, P21 and adulthood. Significant PER2::LUC circadian rhythms were detected at all ages examined in the control, but evident only during the neonatal period (P1 and P7) in Cry1 −/− /Cry2 −/− mice ( Fig. 1b ). Interestingly, the circadian rhythms were not synchronized among littermates in Cry1 −/− /Cry2 −/− mice, which was marked contrast with the well-synchronized circadian rhythms in the control. Similar to Per1-luc , circadian amplitudes increased after birth, peaked at P7–P14 and declined afterwards in the control mice ( Supplementary Fig. S1b ). The amplitude in Cry1 −/− /Cry2 −/− mice was comparable to the control at P1, significantly lower at P7 and P14 and undetectable at P21 and adulthood. A long-term SCN culture confirmed the spindle-like change in circadian amplitude during the early postnatal development in both genotypes ( Supplementary Fig. S1c,d ). The amplitude waxed to a peak around a culture time corresponding to ages P8–P10 (cP8–cP10) and waned thereafter, regardless of whether the SCNs were harvested at P1 or P7. Compared with the control, the circadian amplitude in Cry1 −/− /Cry2 −/− mice was significantly higher at cP6, not different at cP7–cP10 and significantly lower at cP11–cP20 ( Supplementary Fig. S1e ). The circadian period of PER2::LUC rhythm in Cry1 −/− /Cry2 −/− mice was significantly shorter than in the control from cP3 to cP5 but not different thereafter ( Supplementary Fig. S1f ). The exchange of culture medium enhanced the circadian amplitude of PER2::LUC rhythms in the control SCN harvested either at P1 or P21. Medium exchange enhanced circadian amplitude in the Cry1 −/− /Cry2 −/− SCN harvested at P1, but failed to restore the circadian rhythm in the SCN harvested at P21, despite a substantial increase in the basal bioluminescence level ( Supplementary Fig. S2a,b ). Forskolin administration also failed to elicit a circadian rhythm in the SCN of Cry1 −/− /Cry2 −/− mice harvested at P21 ( Supplementary Fig. S2c ). Circadian rhythms in Per1-luc and PER2::LUC were detected at the single-cell level in the SCN of Cry1 −/− /Cry2 −/− mice harvested at P2-P5 ( Supplementary Fig. S2d,e ). The circadian rhythms were disordered and poorly synchronized to each other in Per1-luc , whereas the rhythms were robust and well synchronized in PER2::LUC. Cell morphology in the Cry1 −/− /Cry2 −/− SCN was indistinguishable from that in the control culture harvested from adult and P7 mice. Neither the density of neurons nor the cell shape was different ( Supplementary Figs S3 and S4 ). Circadian rhythms in spontaneous firing in SCN slices To confirm circadian rhythms with a functional measure in addition to the gene expression, spontaneous firing in single neurons of neonatal Cry1 −/− /Cry2 −/− SCN slices were continuously measured for at least 10 days on a MED ( Fig. 2 and Supplementary Fig. S5 ). χ 2 periodogram revealed significant circadian rhythms ( P <0.01) in all neurons examined from the control and Cry1 −/− /Cry2 −/− mice ( Fig. 2b ). The circadian rhythms were well synchronized to each other in both genotypes ( Fig. 2d and Supplementary Fig. S5d ), and the synchronization was kept in Cry1 −/− /Cry2 −/− mice, even when the circadian period abruptly changed ( Fig. 2g ). 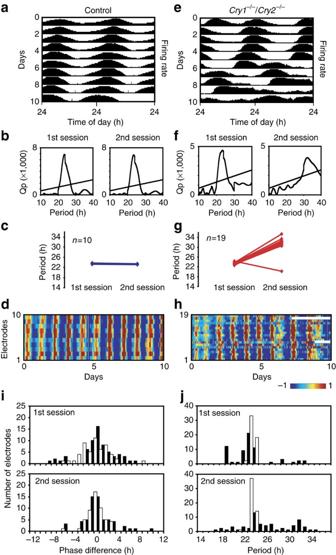Figure 2: Coherent circadian rhythms in spontaneous firing of neonatal SCN slices. Representative circadian rhythms in spontaneous firing are shown for a control (a) and aCry1−/−/Cry2−/−slice (e). Data are double plotted along thexaxis (48-h scale). Firing rate is expressed relative to the maximum value of a series record (percentile histogram; ClockLab).χ2periodograms (b,f) demonstrate significant circadian rhythms in both genotypes and a sudden change in circadian period in theCry1−/−/Cry2−/−slice. An oblique line in the periodogram indicates the significance level (P<0.01). Synchrony of the cellular rhythms measured simultaneously from the same SCN slices is illustrated by the clustering of circadian periods measured for 5 days before (first session) and after (second session) the change of periodicity (c,g). Individual circadian profiles are illustrated in raster plots to show this intercellular synchrony (d,h). SeeSupplementary Methodsfor the details of raster plots. Sample size is indicated on the top of the ordinate. The abscissa indicates the day of analysis. The distributions of circadian phases (i) and periods (j) across single cells from four SCN in the first (upper) and the second sessions (lower) are shown for the control (open column) andCry1−/−/Cry2−/−cells (filled column). The phase distribution was standardized by plotting individual circadian peaks around the slice mean, indicated as the zero value. InCry1−/−/Cry2−/−mice, the adjusted s.d. of phase distribution was 3.3 h in the first session and 2.9 h in the second, which was not significantly different. The circadian period was significantly longer in the second session (mean±s.d.; 26.1±4.5 h,n=61) than the 1st (23.2±3.5 h,n=64), but the adjusted s.d. of period did not change. The adjusted s.d. of circadian phase and period distribution in both sessions were much larger inCry1−/−/Cry2−/−mice than in the controls. These SCN slices were harvested at P2–5. Figure 2: Coherent circadian rhythms in spontaneous firing of neonatal SCN slices. Representative circadian rhythms in spontaneous firing are shown for a control ( a ) and a Cry1 −/− /Cry2 −/− slice ( e ). Data are double plotted along the x axis (48-h scale). Firing rate is expressed relative to the maximum value of a series record (percentile histogram; ClockLab). χ 2 periodograms ( b , f ) demonstrate significant circadian rhythms in both genotypes and a sudden change in circadian period in the Cry1 −/− /Cry2 −/− slice. An oblique line in the periodogram indicates the significance level ( P <0.01). Synchrony of the cellular rhythms measured simultaneously from the same SCN slices is illustrated by the clustering of circadian periods measured for 5 days before (first session) and after (second session) the change of periodicity ( c , g ). Individual circadian profiles are illustrated in raster plots to show this intercellular synchrony ( d , h ). See Supplementary Methods for the details of raster plots. Sample size is indicated on the top of the ordinate. The abscissa indicates the day of analysis. The distributions of circadian phases ( i ) and periods ( j ) across single cells from four SCN in the first (upper) and the second sessions (lower) are shown for the control (open column) and Cry1 −/− /Cry2 −/− cells (filled column). The phase distribution was standardized by plotting individual circadian peaks around the slice mean, indicated as the zero value. In Cry1 −/− /Cry2 −/− mice, the adjusted s.d. of phase distribution was 3.3 h in the first session and 2.9 h in the second, which was not significantly different. The circadian period was significantly longer in the second session (mean±s.d. ; 26.1±4.5 h, n =61) than the 1st (23.2±3.5 h, n =64), but the adjusted s.d. of period did not change. The adjusted s.d. of circadian phase and period distribution in both sessions were much larger in Cry1 −/− /Cry2 −/− mice than in the controls. These SCN slices were harvested at P2–5. Full size image The features above were confirmed in four SCN slices for each genotype. As the circadian period changed abruptly in all four Cry1 −/− /Cry2 −/− slices examined, we separately analysed rhythms before (first session) and after (second session) the period change. In the control slices, corresponding records at analogous times into culture were separately analysed. The phase-adjusted distribution of circadian peaks was not significantly different between the first and second sessions in Cry1 −/− /Cry2 −/− mice, though the distribution of circadian period was shifted to a longer range ( Fig. 2i ). The variability, in terms of s.d., of circadian phase and period was only slightly larger in Cry1 −/− /Cry2 −/− than in the control mice. Circadian amplitude was essentially the same in the control and Cry1 −/− /Cry2 −/− mice. Simultaneous determination of gene expression and firing The circadian rhythms in Per1-luc and PER2::LUC were substantially different at the SCN tissue level in Cry1 −/− /Cry2 −/− mice. To determine whether the differences were due to technical issues or to the intrinsic nature of the circadian rhythms, Per1-luc or PER2::LUC bioluminescence at the cell level were measured simultaneously with spontaneous firing as a reference in the same neonatal SCN slice ( Fig. 3 ). 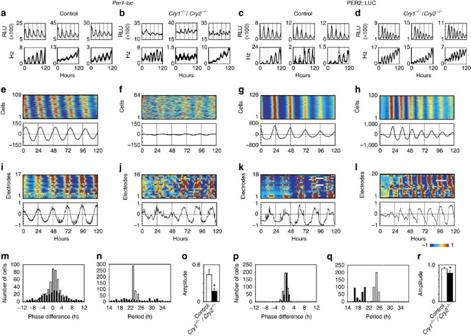Figure 3: Simultaneously determined cellular circadian rhythms in clock gene expression and spontaneous firing in neonatal SCN slices. Representative cellular rhythms inPer1-lucand PER2::LUC bioluminescence (upper panels) fromCry1−/−/Cry2−/−SCN (b,d) and the respective controls (a,c) are shown above the simultaneously recorded spontaneous firing rhythms (lower panels) from the same SCN. Circadian phases in individual rhythms are illustrated (e–l) as raster plots (upper) with mean group profiles (lower). The abscissa of raster plots indicates the time in hours from the midnight (0000 hours in local time) of the day of SCN harvest. A group profile is indicated as the detrended rhythm of bioluminescence obtained from the entire SCN (e–h) and as the averaged values of standardized individual firing rhythms (−1 to +1) (i–l). The distributions of circadian phase (m,p) and period (n,q) in cellular rhythms from three SCN are demonstrated for the controls (open column) andCry1−/−/Cry2−/−mice (filled column). The adjusted s.d. of phase distribution forPer1-lucrhythm was significantly larger inCry1−/−/Cry2−/−mice (4.6 h) than in the controls (2.6 h), but it was not the case for PER2::LUC rhythm (0.7 h versus 0.8 h). The circadian amplitude (o,r) was significantly lower inCry1−/−/Cry2−/−than in the control mice for bothPer1-luc(control:n=438,Cry1−/−/Cry2−/−:n=287) and PER2::LUC (control:n=369,Cry1−/−/Cry2−/−:n=295) rhythms (*P<0.01 versus controls, Mann–WhitneyU-test). All data are given as the mean±s.d. These SCN slices were harvested at P2–5. Figure 3: Simultaneously determined cellular circadian rhythms in clock gene expression and spontaneous firing in neonatal SCN slices. Representative cellular rhythms in Per1-luc and PER2::LUC bioluminescence (upper panels) from Cry1 −/− /Cry2 −/− SCN ( b , d ) and the respective controls ( a , c ) are shown above the simultaneously recorded spontaneous firing rhythms (lower panels) from the same SCN. Circadian phases in individual rhythms are illustrated ( e – l ) as raster plots (upper) with mean group profiles (lower). The abscissa of raster plots indicates the time in hours from the midnight (0000 hours in local time) of the day of SCN harvest. A group profile is indicated as the detrended rhythm of bioluminescence obtained from the entire SCN ( e – h ) and as the averaged values of standardized individual firing rhythms (−1 to +1) ( i – l ). The distributions of circadian phase ( m , p ) and period ( n , q ) in cellular rhythms from three SCN are demonstrated for the controls (open column) and Cry1 −/− /Cry2 −/− mice (filled column). The adjusted s.d. of phase distribution for Per1-luc rhythm was significantly larger in Cry1 −/− /Cry2 −/− mice (4.6 h) than in the controls (2.6 h), but it was not the case for PER2::LUC rhythm (0.7 h versus 0.8 h). The circadian amplitude ( o , r ) was significantly lower in Cry1 −/− /Cry2 −/− than in the control mice for both Per1-luc (control: n =438, Cry1 −/− /Cry2 −/− : n =287) and PER2::LUC (control: n =369, Cry1 −/− /Cry2 −/− : n =295) rhythms (* P <0.01 versus controls, Mann–Whitney U -test). All data are given as the mean±s.d. These SCN slices were harvested at P2–5. Full size image The circadian rhythms in Per1-luc were less robust in the Cry1 −/− /Cry2 −/− SCN neurons than in the control, whereas the spontaneous electrical firing rhythms were indistinguishable between genotypes ( Fig. 3a ). The raster plots together with the 24-h group profile revealed that the rhythm synchrony was disrupted in Per1-luc ( Fig. 3f ), whereas the synchronization was kept well in spontaneous firing ( Fig. 3j ). Although the mean circadian period of cellular Per1-luc rhythm was not different between the two genotypes (control, 23.5±0.9 h and Cry1 −/− /Cry2 −/− , 24.1±6.2 h, mean±s.d. ), the circadian phase and period of Per1-luc rhythm were distributed more widely, and the circadian amplitude was significantly lower in Cry1 −/− /Cry2 −/− mice than in the control ( Fig. 3m–o ). On the other hand, the circadian rhythms in PER2::LUC and spontaneous firing in Cry1 −/− /Cry2 −/− mice were robust ( Fig. 3d ) and well synchronized in the same SCN, similar to the data in the respective control slices ( Fig. 3g ). Antiphasic circadian rhythms were occasionally detected in spontaneous firing as demonstrated in Figure 3l . Circadian rhythms in both measures were also detected in the neonatal SCN cultured with artificial cerebrospinal fluid ( Supplementary Fig. S6a,b ), excluding the possibility that some factor in the culture media induced the rhythm. As for circadian PER2::LUC rhythms, the phase distribution was comparable to that in the control ( Fig. 3p ), and the amplitude was only slightly suppressed in Cry1 −/− /Cry2 −/− mice ( Fig. 3r ). The mean period of cellular PER2::LUC rhythm was significantly shorter in the Cry1 −/− /Cry2 −/− SCN (17.9±0.3 h) than in the control (24.8±0.4 h) ( Fig. 3q ). Thus, differences in the circadian features between the control and Cry1 −/− /Cry2 −/− mice were also detected at the SCN cell level. The distributions of circadian phase and period in Cry1 −/− /Cry2 −/− cells depended on measure. Circadian phase distribution was wider in the Per1-luc rhythm compared with the electrical firing rhythm ( Supplementary Fig. S7c , adjusted s.d. of phase=4.6 h for Per1-luc and 3.0 h for spontaneous firing, P <0.01). Period distribution was similarly wider (5.5 h for Per1-luc and 3.1 h for spontaneous firing, P <0.01). The relationship of PER2::LUC and spontaneous firing variability was opposite. The phase distribution was significantly narrower in the PER2::LUC rhythms compared with the electrical firing rhythms ( Supplementary Fig. S7d , adjusted s.d. of phase: 0.7 h and 3.1 h for PER2::LUC and spontaneous firing, respectively, P <0.01). Period distribution was likewise narrower for PER2::LUC compared with spontaneous firing (0.3 and 1.1 h, respectively, P <0.01). Notably, similar patterns were detected in the control SCN. The distribution of circadian phase was significantly larger in Per1-luc than in spontaneous firing ( Supplementary Fig. S7a ), whereas the phase distribution was slightly but significantly smaller in PER2::LUC than in spontaneous firing ( Supplementary Fig. S7b ). Cellular circadian rhythms in adult SCN slices A lack of circadian rhythms at the SCN tissue level in adult Cry1 −/− /Cry2 −/− mice could be due to either abolishment or desynchrony of cellular circadian rhythms. To examine these possibilities, 24-h profiles of Per1-luc and PER2::LUC were analysed at the single-cell level in the adult SCN slices of Cry1 −/− /Cry2 −/− ( Fig. 4 ) and the control mice ( Supplementary Fig. S8 ). Significant circadian rhythms were detected in 93% (171/183) of the cells examined for Per1-luc and in 94% (143/152) for PER2::LUC in Cry1 −/− /Cry2 −/− mice. 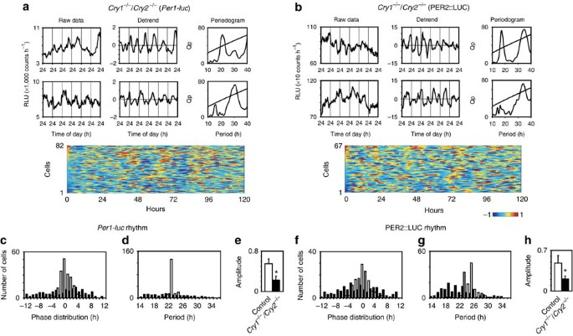Figure 4: Cellular circadian rhythms in adult SCN slices. Representative circadian rhythms in two single cells of an adult SCN slice are expressed as raw bioluminescence (left), detrended records (middle) andχ2periodograms (right) forPer1-luc(a) and PER2::LUC (b) inCry1−/−/Cry2−/−mice. Raster plots of circadian profiles are demonstrated as inFigure 3. The phase and period distributions ofPer1-luc(c,d) and PER2::LUC (f,g) rhythms are illustrated for the control (open column) and forCry1−/−/Cry2−/−mice (filled column). The phase distribution was significantly larger inCry1−/−/Cry2−/−mice (adjusted s.d., number of rhythm-positive neurons/number of neurons examined;Per1-luc, 5.7 h, 171/183 and PER2::LUC, 5.8 h, 143/152) than in the controls (Per1-luc, 1.7 h, 187/187 and PER2::LUC, 2.3 h, 129/129). The period distribution was also significantly larger inCry1−/−/Cry2−/−mice (Per1-luc, 22.2±5.2 h,n=171 and PER2::LUC, 21.6±4.6 h,n=143) than in the controls (Per1-luc, 23.3±1.0 h,n=187 and PER2::LUC, 24.6±1.8 h,n=129). The circadian amplitudes ofPer1-luc(e) and PER2::LUC (h) rhythms inCry1−/−/Cry2−/−mice were significantly lower than those in the respective controls (*P<0.01, Mann–WhitneyU-test). All data are given as the mean±s.d. These SCN slices were harvested from 8- to 12-week-old mice. Figure 4: Cellular circadian rhythms in adult SCN slices. Representative circadian rhythms in two single cells of an adult SCN slice are expressed as raw bioluminescence (left), detrended records (middle) and χ 2 periodograms (right) for Per1-luc ( a ) and PER2::LUC ( b ) in Cry1 −/− /Cry2 −/− mice. Raster plots of circadian profiles are demonstrated as in Figure 3 . The phase and period distributions of Per1-luc ( c , d ) and PER2::LUC ( f , g ) rhythms are illustrated for the control (open column) and for Cry1 −/− /Cry2 −/− mice (filled column). The phase distribution was significantly larger in Cry1 −/− /Cry2 −/− mice (adjusted s.d., number of rhythm-positive neurons/number of neurons examined; Per1-luc , 5.7 h, 171/183 and PER2::LUC, 5.8 h, 143/152) than in the controls ( Per1-luc , 1.7 h, 187/187 and PER2::LUC, 2.3 h, 129/129). The period distribution was also significantly larger in Cry1 −/− /Cry2 −/− mice ( Per1-luc , 22.2±5.2 h, n =171 and PER2::LUC, 21.6±4.6 h, n =143) than in the controls ( Per1-luc , 23.3±1.0 h, n =187 and PER2::LUC, 24.6±1.8 h, n =129). The circadian amplitudes of Per1-luc ( e ) and PER2::LUC ( h ) rhythms in Cry1 −/− /Cry2 −/− mice were significantly lower than those in the respective controls (* P <0.01, Mann–Whitney U -test). All data are given as the mean±s.d. These SCN slices were harvested from 8- to 12-week-old mice. Full size image Raster plots illustrate the desynchronized character of cellular circadian rhythms within the same SCN slice of Cry1 −/− /Cry2 −/− mice ( Fig. 4a ). The distributions of circadian peak phase in both Per1-luc and PER2::LUC on the first culture day were much larger in Cry1 −/− /Cry2 −/− mice than those in the control ( Fig. 4c ). Similarly, the circadian periods of the Per1-luc and PER2::LUC rhythms were distributed widely in Cry1 −/− /Cry2 −/− mice ( Fig. 4d ), which may explain the wide range of phase distribution. The circadian amplitudes of Per1-luc and PER2::LUC rhythms were significantly lower in Cry1 −/− /Cry2 −/− mice than the control ( Fig. 4e ). The cellular circadian rhythms in the Cry1 −/− /Cry2 −/− SCN ( Fig. 4a ) were low in amplitude with superimposed small spikes. They sometimes exhibited a secondary peak in both Per1-luc and PER2::LUC, which could partly be due to a lack of rhythm synchrony. The cellular rhythms could be contaminated by bioluminescence from desynchronized surrounding cells, when the reinforcing effect of SCN cell networks is lost in adult Cry1 −/− /Cry2 −/− mice. However, alteration of the cellular circadian oscillation due to Cry double deficiency is not excluded. Circadian rhythms in isolated SCN cells in dispersed culture The presence of cell-autonomous circadian rhythms and their independence from SCN network properties were further confirmed in dispersed cell cultures of the neonatal SCN from Cry1 −/− /Cry2 −/− mice. Significant circadian rhythms in Per1-luc , PER2::LUC and spontaneous firing were detected in isolated SCN cells at two different cell densities: low cell density (1,100±500 cells mm −2 ) ( Fig. 5a ) and very low cell density (250±80 cells mm −2 ) ( Supplementary Fig. S9 ). Most of the isolated Per1-luc and PER2::LUC positive cells exhibited circadian rhythms, which were indistinguishable in appearance from those in single cells of adult SCN slices from Cry1 −/− /Cry2 −/− mice. The circadian periods of Per1-luc ( Fig. 5c ), PER2::LUC ( Fig. 5e ) and spontaneous firing ( Fig. 5g ) also distributed in a larger range in Cry1 −/− /Cry2 −/− mice than in the control. The circadian amplitudes of Per1-luc and PER2::LUC were significantly lower in Cry1 −/− /Cry2 −/− mice than in the respective control ( Fig. 5d ), but that in spontaneous firing was slightly larger in Cry1 −/− /Cry2 −/− mice than in the control ( Fig. 5h ). 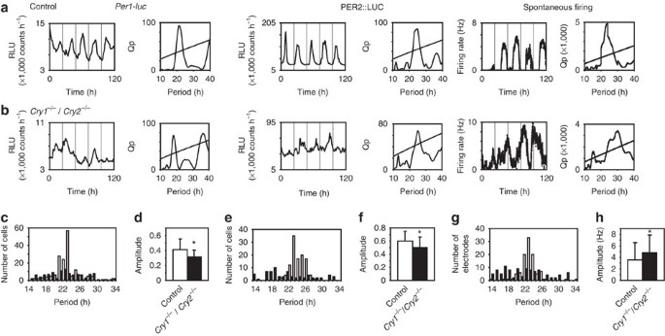Figure 5: Circadian rhythms in isolated cells in dispersed culture of the neonatal SCN. Representative cellular rhythms in dispersed culture of low cell density (ca. 1,100 cells mm−2) of neonatal SCN (n=4–8) from the control (a) andCry1−/−/Cry2−/−mice (b) are shown as measured byPer1-luc(left), PER2::LUC (middle) and spontaneous firing (right), each with corresponding periodograms. Distributions of circadian period are shown (c,e,g) The period distribution was significantly larger inCry1−/−/Cry2−/−mice (open columns,Per1-luc; 22.5±4.7 h,n=111 rhythmic/114 sampled: PER2::LUC; 22.3±5.6 h,n=72/76: firing; 21.3±5.4 h,n=103/104) compared with the controls (filled columns,Per1-luc; 22.7±2.9 h,n=168/168: PER2::LUC; 23.9±1.6 h,n=112/112: firing; 23.1±2.0 h,n=102/104). Significant genotypic effects on amplitude are also shown (d,f,h). (*P<0.01, Mann–WhitneyU-test forPer1-lucand PER2::LUC, Student’t-test for firing). All data are given as the mean±s.d. These dispersed SCN were harvested at P2–5. Figure 5: Circadian rhythms in isolated cells in dispersed culture of the neonatal SCN. Representative cellular rhythms in dispersed culture of low cell density (ca. 1,100 cells mm −2 ) of neonatal SCN ( n =4–8) from the control ( a ) and Cry1 −/− /Cry2 −/− mice ( b ) are shown as measured by Per1-luc (left), PER2::LUC (middle) and spontaneous firing (right), each with corresponding periodograms. Distributions of circadian period are shown ( c , e , g ) The period distribution was significantly larger in Cry1 −/− /Cry2 −/− mice (open columns, Per1-luc ; 22.5±4.7 h, n =111 rhythmic/114 sampled: PER2::LUC; 22.3±5.6 h, n =72/76: firing; 21.3±5.4 h, n =103/104) compared with the controls (filled columns, Per1-luc ; 22.7±2.9 h, n =168/168: PER2::LUC; 23.9±1.6 h, n =112/112: firing; 23.1±2.0 h, n =102/104). Significant genotypic effects on amplitude are also shown ( d , f , h ). (* P <0.01, Mann–Whitney U -test for Per1-luc and PER2::LUC, Student’ t -test for firing). All data are given as the mean±s.d. These dispersed SCN were harvested at P2–5. Full size image TTX desynchronizes cellular circadian rhythms in neonate SCN The contribution of synaptic interaction to the coupling of cellular circadian rhythms was examined in cultured neonatal SCN by TTX application. Although the rhythm amplitude was substantially decreased, significant circadian rhythms in PER2::LUC were observed in single cells of the SCN during TTX treatment in Cry1 −/− /Cry2 −/− mice and in the control ( Fig. 6a–d ). Cellular circadian rhythms under TTX were noisy and desynchronized to each other in Cry1 −/− /Cry2 −/− mice ( Fig. 6e ). These features were similar to the cellular rhythms observed in adult slice or in neonatal dispersed cell cultures of the Cry1 −/− /Cry2 −/− SCN ( Figs 4 and 5 ). The circadian period was much shorter and distributed more widely in Cry1 −/− /Cry2 −/− mice (20.5±5.0 h, n =101) than in the control (24.1±1.2 h, n =140) ( Fig. 6e ). 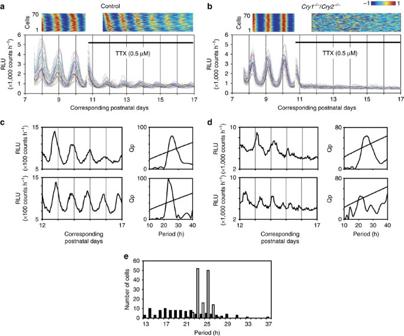Figure 6: Desynchronization of cellular circadian rhythms in neonatal SCN slice ofCry1−/−/Cry2−/−mice by TTX. PER2::LUC bioluminescence rhythms in single cells of the neonatal SCN slice before and during TTX treatment (below) and the raster plots (above) are shown for the control (a) andCry1−/−/Cry2−/−mice (b). Horizontal black bars indicate the period of TTX application. Representative circadian rhythms in two single SCN cells are illustrated as the raw bioluminescence (left), andχ2periodograms (right) are shown for two SCN cells from the control (c) andCry1−/−/Cry2−/−mice (d). The circadian period of cellular rhythm (e) inCry1−/−/Cry2−/−mice (filled columns) was shorter and distributed more widely than in the controls (open columns).These SCN slices were harvested at P3. Figure 6: Desynchronization of cellular circadian rhythms in neonatal SCN slice of Cry1 −/− /Cry2 −/− mice by TTX. PER2::LUC bioluminescence rhythms in single cells of the neonatal SCN slice before and during TTX treatment (below) and the raster plots (above) are shown for the control ( a ) and Cry1 −/− /Cry2 −/− mice ( b ). Horizontal black bars indicate the period of TTX application. Representative circadian rhythms in two single SCN cells are illustrated as the raw bioluminescence (left), and χ 2 periodograms (right) are shown for two SCN cells from the control ( c ) and Cry1 −/− /Cry2 −/− mice ( d ). The circadian period of cellular rhythm ( e ) in Cry1 −/− /Cry2 −/− mice (filled columns) was shorter and distributed more widely than in the controls (open columns).These SCN slices were harvested at P3. Full size image Circadian rhythms restore in adult Cry1 −/− /Cry2 −/− SCN Whether a diffusible factor(s) in the SCN contributes to the coupling of cellular circadian rhythms in PER2::LUC was investigated by coculture of a non-bioluminescent graft SCN with the host bioluminescent SCN slice. The adult host SCN from Cry1 −/− /Cry2 −/− mice did not exhibit circadian rhythms at the tissue level when cocultured with a graft cortex harvested at P7 ( Fig. 7a ). In contrast, coculture of a graft WT SCN obtained at P1 or P7 restored robust rhythmicity in the mutant host ( Fig. 7a ). Less prominent but significant circadian rhythms were also detected when cocultured with a graft Cry1 −/− /Cry2 −/− SCN obtained at P7 ( Fig. 7b ). Circadian rhythms of low amplitude were detectable in some SCN slices cocultured with graft WT SCN harvested at P14 or P21. The mean circadian amplitude during the coculture was significantly higher with a graft WT SCN harvested at P1 and P7 than that with a graft WT cortex at P7 ( Fig. 7c ). The amplitude decreased substantially with graft WT SCN at P14 and P21 as compared with that at P7. 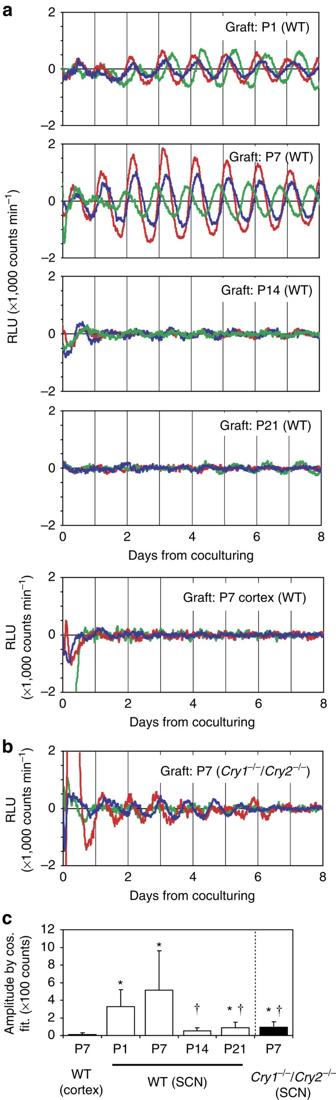Figure 7: Restoration of circadian rhythms in adult SCN slice ofCry1−/−/Cry2−/−mice by coculture of neonatal SCN. Representative PER2::LUC rhythms at the SCN tissue level are shown in adultCry1−/−/Cry2−/−mice expressed by coculture of a graft SCN slice from WT mice at different ages (P1, P7, P14 and P21) (a). Graft cortex slices of WT mice harvested at P7 fail to restore circadian rhythms when cocultured with the adultCry1−/−/Cry2−/−SCN (a). Circadian rhythms of the host adultCry1−/−/Cry2−/−slice were observed in the presence of a P7Cry1−/−/Cry2−/−SCN graft (b). In each panel, different colour traces indicate detrended PER2::LUC bioluminescence of different SCN slices. The circadian amplitude of host SCN, expressed as the amplitude of the best fit cosine curve, was measured from a bioluminescence record of the 3rd to 7th day of coculture (c). The amplitude was significantly higher in the coculture with the P1 (n=4) or P7 (n=7) WT graft SCN compared with coculture with the WT graft cortex (n=4) (*P<0.05, Welch'st-test). The circadian amplitude was also higher in the coculture with the graft SCN ofCry1−/−/Cry2−/−mice (n=5) than in the coculture with the WT graft cortex (*P<0.05, Welch'st-test). Compared with the coculture with the P7 WT graft, the amplitude was significantly lower in the coculture with graft SCN from P14 WT (n=5), P21 WT (n=7) or P7Cry1−/−/Cry2−/−mice (†P<0.05, Welch'st-test). All data are given as the mean±s.d. Figure 7: Restoration of circadian rhythms in adult SCN slice of Cry1 −/− /Cry2 −/− mice by coculture of neonatal SCN. Representative PER2::LUC rhythms at the SCN tissue level are shown in adult Cry1 −/− /Cry2 −/− mice expressed by coculture of a graft SCN slice from WT mice at different ages (P1, P7, P14 and P21) ( a ). Graft cortex slices of WT mice harvested at P7 fail to restore circadian rhythms when cocultured with the adult Cry1 −/− /Cry2 −/− SCN ( a ). Circadian rhythms of the host adult Cry1 −/− /Cry2 −/− slice were observed in the presence of a P7 Cry1 −/− /Cry2 −/− SCN graft ( b ). In each panel, different colour traces indicate detrended PER2::LUC bioluminescence of different SCN slices. The circadian amplitude of host SCN, expressed as the amplitude of the best fit cosine curve, was measured from a bioluminescence record of the 3rd to 7th day of coculture ( c ). The amplitude was significantly higher in the coculture with the P1 ( n =4) or P7 ( n =7) WT graft SCN compared with coculture with the WT graft cortex ( n =4) (* P <0.05, Welch's t -test). The circadian amplitude was also higher in the coculture with the graft SCN of Cry1 −/− /Cry2 −/− mice ( n =5) than in the coculture with the WT graft cortex (* P <0.05, Welch's t -test). Compared with the coculture with the P7 WT graft, the amplitude was significantly lower in the coculture with graft SCN from P14 WT ( n =5), P21 WT ( n =7) or P7 Cry1 −/− /Cry2 −/− mice († P <0.05, Welch's t -test). All data are given as the mean±s.d. Full size image The most striking finding in the present study is that the circadian rhythms in Per1-luc and PER2::LUC at the SCN tissue level damp out during the course of development in Cry1 −/− / Cry2 −/− mice, while the circadian rhythms at the SCN cell level are preserved until adulthood ( Figs 1 and 4 , Supplementary Fig. S1 ). A loss of circadian rhythm at the tissue level is unlikely due to vulnerability to culture of the adult SCN slices, because the SCN of adult Cry1 −/− /Cry2 −/− mice retains the potential to express high-amplitude circadian rhythms. Cellular circadian rhythms were mutually synchronized during the neonatal period but desynchronized after weaning, suggesting that the loss of circadian rhythm at the SCN tissue level is not due to a lack of circadian oscillation but to desynchrony of cellular rhythms from each other. The coherent circadian rhythms expressed in the neonatal Cry1 −/− / Cry2 −/− SCN are subserved by a diffusible factor(s) specific to the neonatal period. CRY1/CRY2 deficiency may interfere with the development of SCN cell networks for rhythm synchrony in adulthood. CRY1 and CRY2 are negative components of the molecular feedback loop for the circadian oscillation [2] , but they are dispensable for the generation of cellular circadian rhythm at least in the neonatal SCN in culture [9] . The roles of CRY1 and CRY2 in the molecular loop could be substituted by other molecules, such as DEC1 and DEC2 [21] , which are known to suppress the E-box-mediated transactivation of Per1 by BMAL1/CLOCK [22] , and the gene expression of which are negatively regulated by PER1 and PER2. They could therefore compensate for the absence of CRY1 and CRY2 in the feedback loop. Alternatively, non-transcriptional mechanisms of circadian oscillation [23] could be involved in a CRY1/CRY2-independent mechanism for rhythm generation. Further studies are needed to elucidate the molecular mechanism of oscillation in Cry1 −/− / Cry2 −/− mice. A loss of circadian rhythm at the SCN tissue level in adult Cry1 −/− / Cry2 −/− mice is most likely due to desynchrony of cellular circadian rhythms in the SCN ( Fig. 4 ). Cellular couplings responsible for rhythm synchrony are mediated by either synaptic communication or autocrine–paracrine mechanisms [9] , [11] that not only synchronize but also reinforce the cellular circadian rhythms [13] . Importantly, the cellular rhythms in the adult Cry1 −/− / Cry2 −/− SCN slice were remarkably similar in appearance and period distribution to those in the dispersed cell cultures or in the TTX-treated SCN slices from neonatal Cry1 −/− / Cry2 −/− mice ( Figs 4 and 5 ), in which cellular coupling is substantially disrupted. Such large period variability was not observed in the control mice. In addition, the circadian period of neonatal SCN in Cry1 −/− / Cry2 −/− mice was significantly shorter than in the control ( Fig. 3 and Supplementary Fig. S1 ). These findings indicate that the cellular circadian rhythms are also affected to some extent by CRY double deficiency. Coculture of neonatal SCN from WT mice restored the circadian rhythm of PER2::LUC in the adult Cry1 −/− / Cry2 −/− SCN ( Fig. 7 ). Less robust circadian rhythms were also restored by coculturing with the SCN harvested at P7 from Cry1 −/− / Cry2 −/− mice. These findings indicate that the cell networks for rhythm synchrony still exist in the SCN of adult Cry1 −/− / Cry2 −/− mice and are capable of expressing the circadian rhythms at the tissue level in response to a diffusible factor(s) in the neonatal SCN. Importantly, the rhythm was not fully restored by older WT SCN grafts, suggesting that the diffusible factor(s) is lost or loses its potency as the SCN develops. Therefore, a loss of coherent circadian rhythms in the adult Cry1 − / − / Cry2 − / − SCN is due to a failure of development of cell networks, which subserve rhythm synchrony without the neonate specific diffusible factor(s) in the SCN. Thus, CRY1/CRY2 are most likely involved in the development of adult type cell networks. The switch from CRY1/CRY2-independent to -dependent cell networks takes place at around P14—P21 ( Supplementary Fig.S10 ). The neonatal SCN from Cry1 −/− / Cry2 −/− mice was less effective in restoring rhythms in host SCNs, suggesting that the putative diffusible factor(s) is less effective compared with WT slices. CRY1/CRY2 may also be involved in the function of this diffusible factor(s). Several molecules have been suggested to mediate cellular coupling in the SCN. The SCN was shown to respond to an agonist of D1 dopamine receptors only during the early postnatal period [24] . Vasoactive intestinal polypeptide was reported to be involved in the cellular coupling of SCN [25] . However, the roles of CRY1 and CRY2 in the dopamine and vasoactive intestinal polypeptide signalling are not known in the SCN. Recently, a new role for CRY1 was proposed in the mouse liver, where CRY1 suppressed the action of adenylate cyclase by interrupting the association of Gs proteins [26] . This is a possible mechanism which links CRY double deficiency to a failure of development of cell networks for synchronized rhythm expression in the adult SCN. Substantial differences in the circadian rhythms were observed between Per1-luc and PER2::LUC at both the cell and tissue levels ( Figs 1 and 3 and Supplementary Fig. S7 ). These differences are unlikely to be due to the difference in the reporter system used. This is because in the control mice, the developmental changes are essentially the same for both measures, whereas in Cry1 −/− /Cry2 −/− mice, several features of the circadian rhythm, such as the amplitude and distribution of phase and period, differed between them ( Supplementary Fig. S1a,b and Fig. 3 ). Circadian rhythms in Per1-luc seem to be more sensitive to CRY double deficiency than those in PER2::LUC. Furthermore, the phase distribution was different even in the control SCN between Per1-luc and PER2::LUC rhythms, which suggest the intrinsic nature of circadian rhythms is different between them. Parameters of the circadian rhythm in spontaneous firing were more similar to PER2::LUC than to Per1-luc rhythms in both genotypes ( Fig. 3 ). The firing pattern of the SCN neuron was reported to differ between the cells which expressed Per1-GFP and those which did not [27] . These findings suggest that the cell networks of the SCN differ for the cell populations expressing Per1-luc and PER2::LUC. Different cell networks may build-up different regional pacemakers of different function as suggested previously [28] . We conclude that the cellular couplings that are responsible for the expression of coherent circadian rhythms differ in the neonatal and adult SCN in mice. The cellular couplings for rhythm synchrony are relatively independent of CRY1/CRY2 in the neonatal SCN, whereas dependent on these molecules in the adult SCN. CRY1/CRY2 is involved in the development of cell networks from the neonatal type to the adult. Animals Cry1 −/− /Cry2 −/− mice were acquired from the Tohoku University [29] , and bred with Per1-luc mice carrying a Per1 luciferase reporter [30] or PER2::LUC mice carrying a PER2 fusion luciferase reporter [31] . They were backcrossed with C57BL/6J mice for more than 13 generations. Cry1 +/+ /Cry2 +/+ Per1-luc transgenic mice [29] and Cry1 +/+ /Cry2 +/+ PER2::LUC knock-in mice [31] on the C57BL/6J background were used as the control. For the measurement of bioluminescence, the transgenic mice were used without discrimination between the homozygote and heterozygote. Although the intensity of the bioluminescence in the homozygote was approximately twice as high as that in the heterozygote, the circadian amplitudes of bioluminescent rhythms were standardized (see data analyses section), and no difference was observed in the standardized circadian amplitudes between the two genotypes. Mice were reared in our animal quarters where environmental conditions were controlled (lights-on 0600–1800 hours; light intensity ~100 lx at the bottom of cage; humidity 60±10%). Cry1 −/− /Cry2 −/− mice were born to Cry1 −/− /Cry2 −/− parents and were raised by their original mother. Both male and female mice were used. The day of birth was designated as the postnatal day 0 (P0). Animals were euthanized to harvest the SCNs between 0800 and 1600 hours. Experiments were conducted in compliance with the rules and regulations established by the Animal Care and Use Committee of Hokkaido University under the ethical permission of the Animal Research Committee of Hokkaido University (approval no.08-0279). SCN slice culture Per1-luc and PER2::LUC bioluminescence at the SCN tissue level was measured with a photomultiplier tube (Actimetrics: Lumicycle). Coronal SCN slices of 300 μm were made with a tissue chopper (Mcllwain) from mice harvested at P1 or P7, and with a DSK Microslicer (DTK-1000; Dosaka EM) from mice harvested at P14, P21, or adult (8–16 weeks old). The SCN tissue was dissected at the mid rostrocaudal region and a paired SCN was cultured on a Millicell-CM culture insert (Millipore Corporation) as previously reported [30] . In coculture experiments, 200-μm-thick SCN slices were obtained from adult Cry1 −/− /Cry2 −/− mice carrying the PER2::LUC reporter and precultured for 4 or 5 days. Bioluminescence was continuously monitored using a photomultiplier tube (Atto: Kronos). Graft was prepared from mice without the reporter system. Graft SCN slices of 200 μm were obtained from the control mice of different ages (P1, P7, P14 and P21) or from Cry1 −/− /Cry2 −/− mice at P7. The graft SCN was precultured for one day before coculturing. A cortex slice from the control mice at P7 was also used as a graft. The host SCN was cocultured with the graft tissue by turning over the graft and laying it on top of the host SCN. The bioluminescence was continuously measured for at least 14 days. Per1-luc or PER2::LUC bioluminescence at the single SCN cell level was measured with an EMCCD camera (ImagEM, Hamamatsu photonics; iXol, Andor). Coronal slices of 200 μm were prepared from neonates with a tissue chopper and those of 100 μm from adults with a microslicer. The SCN tissue was cultured as previously reported, [30] except for the concentration of D-Luciferin K (0.5 mM). TTX (treated 1/100 dilution of 50 μM, final concentration: 0.5 μM) was applied on the culture day corresponding to the postnatal day 10th (cP10) with fresh medium. The spontaneous firing was measured by a MED system. Coronal brain slices of 200 μm thickness were obtained from 2- to 5-day-old pups using a tissue chopper. An SCN slice was placed on a collagen precoated MED and cultured as previously described [32] . Half of the culture medium was exchanged every day for the first several days of culturing and then every second day thereafter. The culture medium was not exchanged during the recording period except where indicated ( Supplementary Fig. S2 ). Dispersed SCN cell culture Four to eight paired SCNs from 2- to 5-day-old pups were dissected from coronal hypothalamic slices of 400 μm thick and then treated together with trypsin as described previously [32] . Dispersed cells were plated on a 35-mm Petri dish or a MED precoated with 0.01% poly- L -ornithine in very low cell density (250±80 cells mm −2 ) or in low cell density (1,100±500 cells mm −2 ). Dispersed cells were plated on 1–3 dishes for the former and on a single dish for the latter. Medium composition was the same as that for the slice culture except for supplementation with 5% fetal bovine serum. Cell dispersion was performed twice for each cell density in both genotypes. The numbers of animals used for culture in the present study are summarized in Supplementary Table S1 . Bioluminescence recording Bioluminescence at the SCN tissue level was measured by a photomultiplier (Lumicycle; Actimetrics) at 10-min intervals with an exposure time of 1 min in a single run of 10–30 days, as previously described [30] . The intensity of bioluminescence was expressed in relative light units (counts per min). Bioluminescence at the SCN cell level in cultured slices or in dispersed cells was obtained by DM IRB (Leica), Luminoview 200 (Olympus) or Cellgraph (Atto) equipped with an EMCCD camera cooled at −80 °C. Bioluminescence was measured every 60 min with an exposure time of 59 min for 7–14 days. The pixel size was 2.3 × 2.3 μm for DM IRB, 2.0 × 2.0 μm for Luminoview 200 and 1.6 × 1.6 μm for Cellgraph. Bioluminescence signals were analysed in terms of a region of interest (ROI). A single SCN cell was identified according to the following criteria: (1) the size of ROI corresponded to the typical SCN neuron (the diameter was ~10 μm), (2) the shape of ROI was round, (3) there was only one highlighted area in the ROI. The mean area of a single ROI measured was about 100 μm 2 , almost equivalent to a single SCN cell. The intensity of bioluminescence was expressed as an average intensity of pixels involved in a ROI. Simultaneous recording of spontaneous firing and bioluminescence Spontaneous firing was recorded for 7–18 days using a MED 64 system (Alpha MED Scientific). The MED with small electrodes (20 × 20 μm; MED-P210A) was used for the SCN slice culture and that with large (50 × 50 μm; MED-P515A) for the dispersed cell culture. Spike discharges with signal–noise ratio >2.0 were collected by Spike Detector software (Alpha MED Scientific) as previously described [33] . The number of spikes per min was calculated for each electrode covered by aSCN slice. The SCN slice of a 2- to 5- day-old pup was cultured on a MED, which was placed in a mini-incubator installed on the stage of a microscope (ECRIPSE TE2000-U, ECRIPSE E1000, Nikon). The culture conditions were the same as those described previously [32] , except that they were performed in 100% air. In some SCN slices, PER2::LUC bioluminescence and spontaneous firing were simultaneously recorded while culturing with artificial cerebrospinal fluid containing 0.1% D -glucose and 0.5 mM D -luciferin K. Bioluminescence was recorded with a CCD camera (ORCA-II, Hamamatsu Photonics) cooled at −60 °C. The pixel size was 4.3 × 4.3 μm. Data analysis Bioluminescence signals from single cells were analysed using Aquacosmos software (Hamamatsu Photonics) or Cellcycle (Actimetrics) as previously described [30] . Bioluminescence records of the first 12 h were excluded from the rhythm analysis because of extremely high initial levels of bioluminescence. The raw bioluminescence data were smoothed using a three-point moving average method. The bioluminescence data and firing records were detrended by a 24-h running average subtraction method. The significance of a circadian rhythm was evaluated by a χ 2 periodogram (ClockLab). A χ 2 periodogram was applied for a record of 5 consecutive days in a period range between 10.0 and 40.0 h, with a significance level of P <0.01. When more than one significant peak was detected in a χ 2 periodogram, a cosine curve fitting method was performed to select the fundamental frequency and exclude the harmonics ( Supplementary Fig. S11 ). The significance of curve fitting was evaluated with the percent rhythm analysis ( P <0.05). Cosine curve fitting was also applied to test the existence of circadian rhythm or to estimate the mean circadian amplitude of successive rhythms in the SCN tissue. Significance of curve fitting was evaluated with a 99% confidence ellipse [34] . Circadian peak was determined by a modified method of Inagaki et al [30] . Circadian amplitude was calculated by subtracting the circadian trough value from the peak in a cycle. In the case of bioluminescence, the circadian amplitude was further standardized by dividing the circadian peak value to eliminate possible slice biases, as the peak–trough difference correlated strongly with the peak level ( r =0.98). In single-cell rhythms, the maximum amplitude of a time series record was selected as the circadian amplitude. The range of distribution (s.d.) in single cells from multiple SCN slices was calculated after eliminating possible slice biases by standardizing the mean value and the number of cells in each slice, because circadian rhythms of the SCN cells in culture were free running and the number of cells analysed was different in each slice. Differences in s.d's were evaluated by F -test. Statistics The group mean is presented as the mean±s.d. T -test or F -test was used when two independent group means were compared, and Mann–Whitney U -test or Welch's t -test was used when the variances of two group means were different. A one-way analysis of variance with a post-hoc Tukey–Kramer test or multiple t -test was applied to a single time series data. A two-way analysis of variance was adapted when two independent time series data were compared (Statview or Statcel 3). How to cite this article: Ono, D. et al . Cryptochromes are critical for the development of coherent circadian rhythms in the mouse suprachiasmatic nucleus. Nat. Commun. 4:1666 doi: 10.1038/ncomms2670 (2013).